Spatio–spectral structures in high-order harmonic beams generated with Terawatt 10-fs pulses A large international effort is nowadays devoted to increase the energy of the extreme ultraviolet pulses by using high-peak power ultrashort fundamental pulses (Terawatt level). Using such fundamental pulses brings specific constraints that need to be addressed. Here we study high-order harmonic generation in gases with 10 fs pulses at Terawatt peak power and demonstrate that extreme ultraviolet beams can be highly structured and complex in various conditions. We use a single-shot spatially resolved spectral detection and demonstrate direct observation of the spatio–temporal coupling occuring in the generating medium. Clear and reproducible complex spatio–spectral structures are observed in the far field. Similar structures are reproduced with simulations and we show that they are intimately associated to the high nonlinearity of high-order harmonic generation. Those findings are of prime importance for the generation of high-energy attosecond pulses and reveal important issues for their applications. High-order harmonic generation (HHG) in gases has opened new domains as the extreme ultraviolet (XUV) beams have specific properties [1] , [2] , [3] like short duration down to the attosecond level [4] , [5] and good spatial coherence [6] . Using high-energy ultrashort laser pulses to generate attosecond pulses in gases is now largely studied as it should provide high-energy attosecond pulses [7] suitable for XUV induced nonlinear processes [8] , [9] and coherent XUV imaging [10] , [11] . When the duration of those high-energy pulses is limited to few cycles, they can efficiently generate high energy isolated attosecond pulses (IAPs) which is nowadays a major concern in Attoscience [9] , [12] , [13] , [14] , [15] , [16] , [17] , [18] . However, using such high-energy fundamental pulses brings specific constraints that need to be addressed and can reveal unexpected behaviour as demonstrated in this work. The XUV spectrum and beam profile provide information on the HHG process itself and on the generating medium [19] , [20] . When the XUV spectra exhibit interferences, it allows to retrieve even more information on the laser–matter interaction [21] . They are therefore major issues in Attoscience and they have been widely studied. Structures due to interferences have been observed in the XUV spectra, and depending on the experimental conditions, they originate from different phenomena: quantum path interference (QPI) [22] , [23] , [24] , [25] , phase matching [26] or caustics [27] . Also, spectral interferences can be observed in the harmonic spectra when the attosecond pulse train is very short [28] , [29] . It is due to the half cycle periodicity of the HHG process that the attosecond pulses of the train interfere with each other and spectral structures related to the number of pulses in the train can appear. In addition, spectral splitting in the harmonic spectra due to the microscopic response [30] or due to propagation in the medium [31] , [32] has also been reported. In this article, we report and study complex structures within individual harmonics originating from a different process than the ones cited above. The spatio–spectral interferences appear directly in the spatially resolved measured spectra and exhibits patterns unobserved so far. Therefore, it provides new informations on the generating process. Here we show that spatio–temporal coupling occurring in the generating medium [33] , [34] can have a dramatic contribution in the spatio–spectral interference patterns in the far field even without propagation or phase-matching considerations and even with a single quantum path contribution. This work is performed in the context of the large international effort devoted to the development of Terawatt (TW) level laser facilities to obtain and control intense attosecond pulses. The observed harmonics consist of short train of attosecond pulses with large spectra that can even get continuous. Those observations are also important for the attoscience field because the conditions used here to generate the harmonics are similar to those providing high-energy IAP [16] , [17] . We focus on plateau harmonics in this study as these harmonics are more efficiently generated than cutoff harmonics and are potentially interesting for ultra broadband attosecond pulses. We had therefore maximized the harmonics photon number that could be obtained with the constraint of our setup (focal length limited to few metres) for the studied spectral range. In this work, specific experimental parameters (high-energy 10-fs pulses and long focal length) and the characterization method (single-shot acquisition with high spatial and spectral resolution) enable to reveal structures in the harmonic spectra that have not been observed so far. Note that if such structures were present in previous works, they should be difficult to observe on a multishot basis even with a carrier envelop phase (CEP) stabilized laser system (see Supplementary discussion ). Indeed, the structures are highly dependent on severals parameters such as the pulse temporal profile, the peak intensity, the beam spatial profile, the CEP of the pulse. Thus, small pulse-to-pulse fluctuations that are inherent to a laser chain could rule out their contrast making them unobservable when the detection is averaged over several shots (see Supplementary Figs 1,2 ). To finely investigate those phenomena, we performed systematic studies to characterize a harmonic beam emitted by a high-energy ultrashort pulse with high spectral and spatial resolution on a single-shot basis. We used TW ultrashort laser pulses (10 mJ, 10 fs) provided by an ionization-based postcompression technique [35] , [36] , [37] . Those ultrashort driving pulses are loosely focused into an argon gas jet. Note that with TW beam, thin media are better fitted than long media for HHG. Indeed, the propagation of high-peak power beams (above the critical power for self-focusing) over long distances would be complex and this would make the understanding and control of the HHG beam difficult. The ultrashort TW pulses allowed us to obtain broad harmonics (up to a continuum) and to observe well-resolved spectral interference patterns. The single-shot acquisition allows overcoming fluctuation issues of the driving pulses and gives access to instantaneous measurement of physical quantities instead of averaged values. In our conditions, we observed highly structured spectra in strong contrast to the smooth spectra commonly reported using high-energy few-cycle pulses [16] , [38] , [39] . In this article, we give a deeper insight of the underlying process involved in the generation of high-energy attosecond pulses and address issues related to the time-dependent shape of the harmonic source. Attosecond XUV pulses have a complex space–time structure and the temporal characterizations that are spatially averaged do not enable to retrieve this complex structure. The spatial properties of HHG has already been investigated using two-colour laser field [40] , [41] and this method has been recently used to perform space–time characterization of attosecond pulses [42] . Here we show that the space–time coupling involved in HHG is directly encoded in the harmonic spectrum and that the detection method using high spatial and spectral resolution on a single-shot basis enable to investigate space–time characteristics of the XUV emission in the near field. This method gives access to spatio–temporal beam homogeneity in the far field and provide therefore a way to optimize the uniformity of the generating process. It would allow the production of spatially uniform and high contrast attosecond pulses at high energy level. Experimental observations We first investigated the influence of the intensity and interaction geometry on the spatially resolved harmonic spectra by aperturing the fundamental beam with an iris located before the focusing mirror (see the influence of the iris diameter φ iris , Supplementary Fig. 3 ). The Fig. 1 presents spatially resolved single-shot harmonic spectra for several iris diameters. The output of the nozzle is placed very close to the laser beam to limit the expansion of the medium before interaction and thus generate the harmonics in a very thin medium (much thinner than the confocal parameter) but in a large volume ( w 0 >115 μm). For the spectra presented in Fig. 1 , the impact of propagation in the medium is therefore minimized and the beam characteristics is mainly imposed by the spatial coherence of the source. 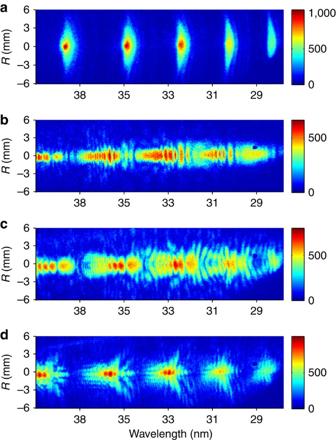Figure 1: Spatially resolved single-shot harmonic spectra generated in argon. The backing pressure of the gas jet isPAr=4.5 bar. The gas jet is placed 5 cm before focus. The intensity in the generating mediumIIRdepends on this iris diameterφiristhat clips the beam before focusing. In this range, increasingφirisincreases the intensity and reduces the beam size in the generating medium.ais a reference spectrum with long pulses (HHG with uncompressed fundamental pulseτ=40 fs),φiris=12 mm,IIR=1.2 × 1015W cm−2;b,c,dare generated with 10-fs 10-mJ pulses in a loose focusing regime (f=2 m), 5 cm before the focus (z=−0.43bwithbthe confocal parameter equal to 11.6 cm forφiris=14 mm). Forb,φiris=10 mm andIIR=1.2 × 1015W cm−2; forc,φiris=12 mm andIIR=1.7 × 1015W cm−2; ford,φiris=14 mm andIIR=2.3 × 1015W cm−2. The colour bars are arbitrary units of detected intensity. Figure 1: Spatially resolved single-shot harmonic spectra generated in argon. The backing pressure of the gas jet is P Ar =4.5 bar. The gas jet is placed 5 cm before focus. The intensity in the generating medium I IR depends on this iris diameter φ iris that clips the beam before focusing. In this range, increasing φ iris increases the intensity and reduces the beam size in the generating medium. a is a reference spectrum with long pulses (HHG with uncompressed fundamental pulse τ =40 fs), φ iris =12 mm, I IR =1.2 × 10 15 W cm −2 ; b , c , d are generated with 10-fs 10-mJ pulses in a loose focusing regime ( f =2 m), 5 cm before the focus ( z =−0.43 b with b the confocal parameter equal to 11.6 cm for φ iris =14 mm). For b , φ iris =10 mm and I IR =1.2 × 10 15 W cm −2 ; for c , φ iris =12 mm and I IR =1.7 × 10 15 W cm −2 ; for d , φ iris =14 mm and I IR =2.3 × 10 15 W cm −2 . The colour bars are arbitrary units of detected intensity. Full size image The experimental spectra with the short pulses ( Fig. 1b–d ) exhibit clear and complex spatio–spectral structures that have not been reported so far. The reference spectrum ( Fig. 1a ) obtained with long pulses (40 fs) has a well-known shape with sharp and well-defined harmonics. They are, however, spectrally asymmetric, which is a signature of ionization that restrict emission to the leading edge of the pulse [34] (symmetric harmonics similar to those shown in Heyl et al . [26] could be obtained at lower intensity). With post-compressed 10-fs fundamental pulses ( Fig. 1b–d ), prominent, complex and reproducible structures were observed and consecutive harmonics showed similar structures. For φ iris =10 mm ( Fig. 1b ), we observed a quasi-continuum with clear spectral structures. For φ iris =12 mm ( Fig. 1c ), corresponding to higher intensity in the generating medium, additional spatial structures appeared. While opening the iris further ( φ iris =14 mm, Fig. 1d ), the spatial fringes get more pronounced and more numerous. When the intensity gets too high, the spectral bandwidth of the harmonics decreases ( Fig. 1d ). This could be due to the fact that the XUV emission is restricted to the leading edge of the pulse before the inflection point of the intensity temporal profile that gives the largest spectral shift. Spectral and spatial structures are asymmetric within a harmonic. The spatial fringe spacing is smaller on their red side and larger on their blue side. Similarly, the spectral fringe spacing is very small on the red side and gets larger on the blue side. These structures were robust and qualitatively maintained shot after shot. However, the details could change from one pulse to the next and the structures were washed out by averaging the spectrum over several shots ( Supplementary Fig. 2 ). We also studied the influence of propagation and phase matching on the interference patterns. The Fig. 2 shows harmonic spectra obtained with the same laser parameters but with different interaction conditions (density and length of the generating medium). We were basically changing the distance d jet between the output of the gas jet and the laser propagation axis. The gas jet is not collimated and therefore, the more the distance d jet increases, the more the laser will propagate in a long and diluted medium. Despite the change of the interaction conditions, all the spectra remain highly structured and complex (see Fig. 2 ). The structures get more pronounced in the optimized conditions for high XUV photon flux, when the generating medium is short and dense in our case. Starting from d jet =4 mm ( Fig. 2a , long medium and low pressure), the spatial divergence is low and similar for all wavelengths. The total signal is relatively low but the spectral interferences are already present. For shorter distances ( d jet =2.5 mm, Fig. 2b ), the overall signal is higher and the properties are close to the previous ones ( Fig. 2a ) with a slightly larger XUV beam divergence. The spectral fringes are also very similar even if some details like their position could slightly change. Moving the gas jet from d jet =2.5 mm to d jet =1.3 mm ( Fig. 2b–e ) does not affect significantly the structures, the interference patterns are qualitatively similar. However, the overall signal and the XUV beam divergence are increased. For Fig. 2e ( d jet =1.3 mm), spatial fringes are clearer due to the overall increase of signal and the decreasing influence of propagation. Indeed, for shorter medium, the propagation that tends to filter the off-axis emission is reduced and the spatial fringes can appear clearer. A curvature also appears in the fringes and this implies that there is spatio–temporal coupling during the generation process. For a very short and dense medium ( d jet =0.5 mm, Fig. 2f ), there is much more XUV signal and the divergence gets larger. All the fringes are now curved and the spatial fringes are more pronounced. They are stronger for longer wavelength. However the on-axis spectral interferences still exhibit the same patterns. We also stress that the XUV photon flux is maximum for a short and dense medium, which corresponds to the conditions where the structures are most pronounced. 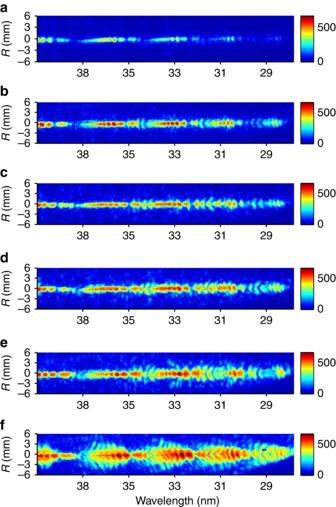Figure 2: Single-shot harmonic spectra for different gas jet radial position. φiris=12 mm, generation in an argon gas jet placed 5 cm before focus,PAr=4.5 bar,djetis the distance between the output of the gas jet and the laser propagation axis. (a)djet=4 mm, (b)djet=2.5 mm, (c)djet=2.2 mm, (d)djet=1.7 mm, (e)djet=1.3 mm, (f)djet=0.5 mm. The intensity is in arbitrary units, however, it allows to compare the detected photon flux as the detection parameters and the colour scale remains unchanged. Figure 2: Single-shot harmonic spectra for different gas jet radial position. φ iris =12 mm, generation in an argon gas jet placed 5 cm before focus, P Ar =4.5 bar, d jet is the distance between the output of the gas jet and the laser propagation axis. ( a ) d jet =4 mm, ( b ) d jet =2.5 mm, ( c ) d jet =2.2 mm, ( d ) d jet =1.7 mm, ( e ) d jet =1.3 mm, ( f ) d jet =0.5 mm. The intensity is in arbitrary units, however, it allows to compare the detected photon flux as the detection parameters and the colour scale remains unchanged. Full size image In conclusion of those experimental studies, these spatio–spectral interferences are highly sensitive on the intensity spatial distribution (profile and amplitude) and changing the iris diameter induces a spectacular evolution in the spatio–spectral coupling of the detected XUV spectra. It implies that the structures are intimately associated to the nonlinearity of HHG. Also, the observation of spatio–spectral coupling in the far-field spectra should intrinsically translate the space–time dependence of the harmonic emission in the near field. In addition, the spatio–spectral features are qualitatively preserved despite the changes of pressure and length of the medium. The structures get more pronounced and the signal is maximized when the generating medium gets short and dense. When d jet is changed, the phase-matching conditions that evolve with density and length of the medium are changed but the spectral structures are present for all the gas jet positions. This implies that the phase matching or the propagation are not the dominant mechanisms creating the observed structures in contrary to previous works [22] , [26] , [31] . Neither QPI, that requires specific interaction conditions to appear [23] , [24] , [25] and strongly changes from one harmonic to the other, is a dominant mechanism here. Spectrally and spatially resolved far-field calculations To investigate numerically those phenomena, we calculated the microscopic response of the target as a function of time and space using the theory described by Strelkov [43] . Being based on the strong field approximation, this theory uses tabulated ionization rates and estimates realistic ratio of the different quantum path contributions in the generation process (for a single atom in the near field). The microscopic response is used to further calculate the macroscopic XUV signal in the far field with the approach described by Platonenko et al . [44] (see Supplementary Method ). Some simulated spectra are presented in Fig. 3 for different conditions approaching the experimental parameters and the spectra are highly structured. For φ iris =10 mm ( Fig. 3a ), the spatio–spectral structures are already clear and the spatial ones are more pronounced than the spectral ones. The bandwidth of the harmonics is smaller than in the experiment, this could be due to different factors. The long path contribution that give a larger spectral broadening seems to be weaker in the far field than in the experiment. If the code gives a realistic ratio of the different quantum path for the microscopic response, the contribution in the far field depends on the macroscopic effect in the near field and therefore on many parameters (driving beam profile and wavefront, temporal pulse profile). For φ iris =12 mm ( Fig. 3b ), the spectral structures get more visible and the spatio–spectral diffraction patterns get very similar to Fig. 1c,d ( φ iris =12–14 mm). And for φ iris =14 mm ( Fig. 3c ), we observed very clear spatio–spectral structures all over the simulated spectra. 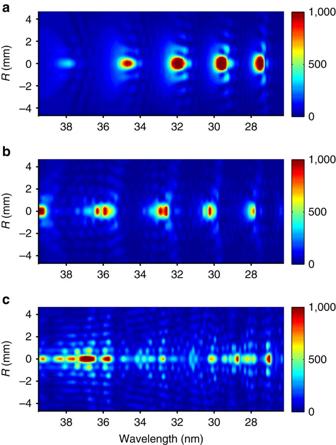Figure 3: Simulated far-field spatially resolved spectra. The driving fieldE0(r,t) in the generating medium 5 cm before focus is calculated by diffracting the beam apertured by an iris of diameterφirisand focused by a 2-m focal length. The beam is assumed perfectly Gaussian before the iris. The input parameters are chosen to approach the experimental conditions: the beam radius atis 10 mm, the pulse energy is 10 mJ and the pulse duration is 10.67 fs with acos2temporal profile (four cycles), the CEP of the pulse is equal to zero. Similar to the experiment, the intensity in the generating mediumIIRdepends onφiris: (a)φiris=10 mm andIIR=1.15 × 1015W cm−2, (b)φiris=12 mm andIIR=1.85 × 1015W cm−2, (c)φiris=14 mm andIIR=2.34 × 1015W cm−2. The propagation is taken into account through modification of the IR wavefront. The length of the medium is 500 μm for an effective pressure of argon of 30 mbar. Figure 3: Simulated far-field spatially resolved spectra. The driving field E 0 ( r , t ) in the generating medium 5 cm before focus is calculated by diffracting the beam apertured by an iris of diameter φ iris and focused by a 2-m focal length. The beam is assumed perfectly Gaussian before the iris. The input parameters are chosen to approach the experimental conditions: the beam radius at is 10 mm, the pulse energy is 10 mJ and the pulse duration is 10.67 fs with a cos 2 temporal profile (four cycles), the CEP of the pulse is equal to zero. Similar to the experiment, the intensity in the generating medium I IR depends on φ iris : ( a ) φ iris =10 mm and I IR =1.15 × 10 15 W cm −2 , ( b ) φ iris =12 mm and I IR =1.85 × 10 15 W cm −2 , ( c ) φ iris =14 mm and I IR =2.34 × 10 15 W cm −2 . The propagation is taken into account through modification of the IR wavefront. The length of the medium is 500 μm for an effective pressure of argon of 30 mbar. Full size image The structures in the simulated spectra are in qualitative agreement with the experiment. They present both spectral and spatial components that evolve with the iris diameter. The calculations allowed to investigate the underlying process driving those structures and to understand the phenomenon. They indicated that the structures are due to the spatial coherence of the emission and its rapid temporal evolution. They can also be obtained with a single quantum path (see Supplementary Figs 4,5 ), which confirm that they are created by a different process than QPI [22] , [23] , [24] , [25] . Note that the fine details of the structures highly depend on several parameters, such as the intensity spatial profile and amplitude (see Supplementary Fig. 5 ), the wavefront of the driving pulses, the pulse temporal profile (see Supplementary Fig. 6 ), the CEP, and so on, and any imperfection of the laser pulses will impact the spectral patterns. For this reason it is difficult to obtain a quantitative agreement between theory and experiment but a qualitative agreement is obtained. The differences could be due to a discrepancy between the experimental beam and the calculated intensity distribution and wavefront of the theoretical beam considered as Gaussian. Also, modification of the fundamental beam profile induced by nonlinear effects during propagation in the medium are not taken into account in the simulations. This approximation is valid for thin medium and low pressure (500 μm and 30 mbar here). However, the modification of the phase of the fundamental (wavefront and instantaneous frequency) due to ionization (main nonlinear effect for the thin medium) are taken into account along the propagation. All linear propagation effects are taken into account for both the fundamental pulses and the harmonics and they have only a minor impact on the structures. We also observed numerically that propagation does not significantly alter the spectral fringes even if it can change the divergence of the XUV beam which is in good agreement with the experimental study in Fig. 2 . Consequently, propagation, phase matching or QPI, in contrary to previous works [22] , [23] , [24] , [25] , [26] , [31] , are not the dominant mechanisms driving the spatio–spectral structures that we observed. The key parameters are the nonlinearity of the atomic response, its saturation and the depletion of the ground state so that the harmonic source is shaped spatially and temporally during the generation process. The time-dependent shape of the harmonic source leads to complex diffraction patterns in the far field. Those patterns therefore originate form self-induced structures in the generating medium. Time- and space-dependent near-field calculations To further analyse these self-interference effects, we investigated the near-field dipole signal as a function of time and space as shown in Fig. 4 . We also investigated the frequency–space domain for each quantum path contribution (see Supplementary Fig. 7 and Supplementary Discussion ). The calculations clearly show that the spatial distribution of the dipole strongly evolves during the pulse on a few femtosecond time scale. Second, the harmonic dipole spatial distribution is clearly not Gaussian and must induce structures in the far field. As shown in the time-integrated plot ( Fig. 4d ), there are two predominant emitting regions that creates the spatial interferences observed in the far field. 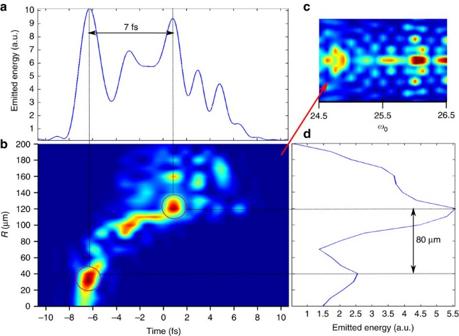Figure 4: XUV emitted intensity in the near field from 24.5ω0to 26.5ω0. This spectral range corresponds to the broadened and blueshifted harmonic 25 and allows to investigate the mechanisms creating the structures in the far field within a harmonic.bnear field XUV emission as a function ofrandt. It corresponds to the spectrum onFig. 2crestricted to the spectral range 24.5ω0–26.5ω0;ais the integrated plot ofbin the spatial dimension,dis the integrated plot ofbin the temporal dimension. Inb, the two dominant dipole emissions in time and space are indicated by red circles. They are separated by 7 fs in the time domain and by 80 μm in the space domain.cis the far field corresponding to the near field presented inbafter 3 m of propagation. a.u., arbitrary unit. Figure 4: XUV emitted intensity in the near field from 24.5 ω 0 to 26.5 ω 0 . This spectral range corresponds to the broadened and blueshifted harmonic 25 and allows to investigate the mechanisms creating the structures in the far field within a harmonic. b near field XUV emission as a function of r and t . It corresponds to the spectrum on Fig. 2c restricted to the spectral range 24.5 ω 0 –26.5 ω 0 ; a is the integrated plot of b in the spatial dimension, d is the integrated plot of b in the temporal dimension. In b , the two dominant dipole emissions in time and space are indicated by red circles. They are separated by 7 fs in the time domain and by 80 μm in the space domain. c is the far field corresponding to the near field presented in b after 3 m of propagation. a.u., arbitrary unit. Full size image Those two predominant regions correspond to emission at two different times, leading to interference in the frequency domain. Therefore, this spatio–temporal coupling creates frequency-dependent spatial structures as observed experimentally and numerically. Note that the emission from the central region should produce an IAP in the near field and this is consistent with the spectral bandwidth in the far field. Nevertheless, the spectrum is modulated everywhere as the near-field off-axis emitters contribute also to the far-field on-axis signal. In the time domain, mainly few (two or three) times of emission are predominant leading to the observation of clear spectral structures. In particular, the main emission times as indicated in Fig. 4a,b are separated by 7 fs. This delay in the emission produces interferences in the frequency domain with an inter-fringe of with q the harmonic order and N t the emission time difference normalized to the infrared (IR) time period, explaining the numerous spectral fringes observed. Note that if the emission was evenly distributed in time, the fringes would have been washed out and despite the long XUV emission (several attosecond pulses) the spectrum would appear continuous. From the spatial point of view, the inter-fringe distance also evolves within a harmonic and as a spectral position can be associated to an emission time [26] , it translates the time evolution of the size of the source: the emission from the rising edge of the IR pulse, corresponding to a smaller size of the emitting region, will correspond to a blueshifted frequency with a large spatial pattern in the far field ( Figs 1d , 3b,c , 4c ). In contrast, the latest emission in Fig. 4 in the falling edge of the pulse corresponds to a red frequency shift and to narrower spatial patterns in the far field due to a bigger size of the emitting region. Therefore, within a harmonic, the spatial patterns should shrink as the wavelength increases as observed in Figs 1d , 3b,c , 4c . The average spatial inter-fringe distance is about 1 mm, which is in good agreement with the expected interference patterns from two sources separated by 80 μm ( with D =3 m and λ =30 nm). Similarly, in the spectral domain, the small fringes are on the red side of the harmonic corresponding to the interference between the broadband emission from the rising edge (one or few attosecond pulses) and the red-shifted emission from the falling edge of the pulse (latest emission) originating from the highest radii where the emission occurs ( Figs 1d , 3c , 4c ). The investigation of the time and space dependence of the harmonic dipole in the near field is therefore consistent with the observed structures in the far field (experimentally and numerically) and the self-interference phenomena that induces them is well understood. However, the near-field spatial distribution of the emitting dipole is surprisingly complicated in this saturation regime. The parabolic shape is consistent with the fact that the XUV yield is stopped early in the pulse leading edge at the centre of the beam due to the fast ionization, while it keeps growing further from the centre of the beam where peak intensity is lower. The dips in the centre and at r =80 μm is due to the complex interplay between the temporal profile, the spatial profile and the CEP of the pulse, which is emphasized by the high nonlinearity of the process and the non-monotonic response on the IR intensity [45] . We experimentally demonstrate HHG with TW ultrashort pulses obtained via an ionization-based post-compression technique. This technique that overcomes the usual energy limitation of self-phase modulation based technique is therefore validated for HHG and it could be a viable solution for large high-energy attosecond facilities that are nowadays being developed. We have studied spatio–spectral structures in the XUV beam generated by HHG in gases and demonstrated that spatio–temporal coupling in the generating medium can lead to observable structures in the far field. We show that these structures are related to the spatial coherence of the harmonic generation process and can be explained for a single quantum path without considering phase matching or propagation effects in the medium (even if they can contribute). Harmonic spectra are the result of numerous coupled physical phenomena, which constitute not only their richness but also their complexity. Specific experimental conditions could promote one mechanism with respect to the others. However, the observation of this self-induced structures can hardly be performed on a multishot basis. Even for a very stable laser system, the inherent fluctuation of the temporal profile, spatial profile and of the CEP would rule out the contrast of the structures. The use of high-energy utrashort pulses on a single-shot basis allowed us to observe those structures clearly by strongly shaping the generating medium but this observation is more general. Such self-interference effects should exist as soon as the atomic response starts to saturate in some part of the XUV source, which induces a different time evolution for the saturating region. This is almost always the case for high-energy harmonic source as the maximum XUV yield is often obtained by saturating some of the emitters and especially when high-energy fundamental pulses are used. It is known that the XUV pulse duration can be strongly lengthened by spatial effects [33] , [34] , [46] . For this reason, spatial filtering are used to select an IAP [47] and it strongly decreases the output energy. However, it appears clearly in our study that even if the emitters are spatially separated in the generating medium, they can all contribute to the XUV emission in the far field. In other words, even if the near-field emission is very short at the centre of the beam, off-axis emitters can also contribute on-axis in the far field and it rules out the possibility of selecting a clean attosecond pulse in our conditions. In addition, we demonstrate that a structured spectrum in single-shot measurement could appear smooth and continuous when averaged over several shots or spatially averaged. Therefore, characterizing the pulse duration with spectrally based measurement techniques would provides inaccurate results. Our observations also question the temporal characterization of attosecond source [48] because the spectrally based techniques rely on the hypothesis of perfect spatial homogeneity of the XUV beam and have been developed in a one-dimensional approach (spatially averaged) [5] , [49] . Therefore, those techniques may be parsimoniously used, when the XUV beams are spatially inhomogeneous, as this may translate in nonrealistic estimations of the pulse duration [46] , [48] , [50] . It points out the importance of finely controlling the intensity distribution in the generating medium for high-energy attosecond pulse generation [15] . Moreover, the generating conditions used in our study are those optimizing the XUV signal. Our detection method would give a way to check the uniformity of the generating process by monitoring the uniformity of the far-field spatially resolved spectra. The method could be coupled with spatial shaping techniques [15] , [51] , [52] to optimize the uniformity of the attosecond pulse in large volume and therefore to allow the production of clean attosecond pulses at high energy level. In addition to the spatial shaping technique, controlling the temporal shape of the pulse via ultrafast pulse shaper that can be integrated in the laser chain would open an excellent way to optimize the attosecond pulses. Indeed, after the CEP control has been widely investigated for attoscience, because those spatio–temporal coupling are very important when generating with high-energy ultrashort pulses, it is now time to investigate an accurate control of both the temporal and spatial profile of the pulse to achieve a novel breakthrough in the field. Postcompression of the driving pulses In this work, the fundamental driving pulses used for HHG are obtained via a postcompression technique that uses self-phase modulation induced by gas ionization in guided geometry [35] . The pulses that seed the hollow-core fibre compressor are supplied by a chirp pulse amplification Ti:Sapphire laser system. Their duration is 40 fs for a carried out energy of 70 mJ at 10-Hz repetition rate. The central wavelength is 810 nm. For the proof of feasibility, we first re-compressed a small fraction of energy (sample beam) [35] . The beam is coupled into a 420-μm inner diameter hollow-core fibre using a 3-m focal length spherical mirror. The fibre is 40 cm long and a very low pressure of helium gas (~10 mbar) is injected through a hole in the cladding located 25 cm from the entrance. The pulses undergo a large spectral broadening as they propagate through the ionizing medium. The spectral bandwidth is increased above 100 nm and the spectra are blueshifted down to 750 nm. The compensation of the chirp at the output of the fibre is performed with chirped mirrors and calibrated silica plates. The shortest pulses have been measured with a second harmonic generation single-shot frequency resolved optical gating (SHG-FROG) and 11.4-fs pulses have been demonstrated on the sample beam for a total output energy of 13.7 mJ [35] , [36] , [37] . For the present experiment, we re-compressed under vacuum the whole output energy of the capillary to use the post-compressed pulses for HHG. The experimental setup of the vacuum compression line and the high-energy attosecond source is presented in Supplementary Fig. 8 . An improvement of the capillary transmission compared with the previous results [35] allowed to use slightly higher pressures of helium and to achieve 10-fs pulses with an output energy of 10 mJ. After optimizing the stability of the system, we obtained a pulse duration fluctuation of 5.6% r.m.s. Shorter pulses (sub-10 fs) could also be obtained with slightly less energy. Supplementary Fig. 9 shows the autocorrelation measurement of the initial pulse and the post-compressed pulses. The FWHM pulse duration is 40 fs for the input pulse, and 10 fs for the post-compressed pulse for an energy of 10 mJ thus reaching a compression factor of 4. It is worth noticing that the autocorrelation trace of the post-compressed pulses are clean and no double pulses or wings appear. Consequently, it rules out the possible contribution of pre-pulses to the observed spectral structures, they are induced by the generating process itself. HHG with TW 10-fs pulses After compression, high-peak power pulses are obtained (10-fs, 10-mJ) which allows for reaching the ionization saturation regime with a loose focusing geometry (10–14 mm diameter beam focused with 2 metre focal length spherical mirror; f −number >140). The experimental setup of the harmonic source is shown in Supplementary Fig. 8b . The intensity distribution (amplitude and shape) at focus is controlled via a motorized iris. The harmonics are generated in an argon gas jet (250-μm cylindrical nozzle) with a backing pressure of 4.5 bar located 5 cm before the beam focus. The gas jet position is z =−0.25 b ( b is the confocal parameter which depends on the iris diameter) for φ iris =10 mm and z =−0.43 b for φ iris =14 mm. Attosecond pulse measurement in the temporal domain has been reported for the latter position and it provided clean attosecond pulses [48] . The peak intensity in the medium is estimated to be 1−2.5 × 10 15 W cm −2 (depending on the iris diameter φ iris ), which is high above the over-barrier intensity in argon ( I OBI =2.47 × 10 14 W cm −2 ; (ref. 53 )). The harmonics are characterized spatially and spectrally using XUV spectrometer equipped with a 500-μm entrance slit located 1.8 m away from the gas jet. The slit is imaged in the spectral dimension using an Hitachi flat field concave grating (1,200 g mm −1 ) onto 40-mm diameter micro-channel plates coupled with a phosphor screen, itself imaged onto a coupled charge device camera. The setup provides spatially and spectrally resolved harmonics measurements. Their spatial profiles are characterized after 3 m of free propagation (the detector is 1.2-m away from the slit). The number of XUV photons is high enough to perform single-shot acquisitions. How to cite this article: Dubrouil, A. et al . Spatio–spectral structures in high-order harmonic beams generated with Terawatt 10-fs pulses. Nat. Commun. 5:4637 doi: 10.1038/ncomms5637 (2014).